Frequency stabilization in nonlinear micromechanical oscillators Mechanical oscillators are present in almost every electronic device. They mainly consist of a resonating element providing an oscillating output with a specific frequency. Their ability to maintain a determined frequency in a specified period of time is the most important parameter limiting their implementation. Historically, quartz crystals have almost exclusively been used as the resonating element, but micromechanical resonators are increasingly being considered to replace them. These resonators are easier to miniaturize and allow for monolithic integration with electronics. However, as their dimensions shrink to the microscale, most mechanical resonators exhibit nonlinearities that considerably degrade the frequency stability of the oscillator. Here we demonstrate that, by coupling two different vibrational modes through an internal resonance, it is possible to stabilize the oscillation frequency of nonlinear self-sustaining micromechanical resonators. Our findings provide a new strategy for engineering low-frequency noise oscillators capitalizing on the intrinsic nonlinear phenomena of micromechanical resonators. Mechanical oscillators are an essential component of practically every electronic system requiring a frequency reference for time keeping or synchronization [1] , [2] , [3] and are also widely used in frequency-shift-based sensors of mass, force, and magnetic field [4] , [5] , [6] , [7] . Currently, micro- and nano-mechanical oscillators are being developed as an alternative to conventional oscillators, such as quartz oscillators, supported by their intrinsic compatibility with standard semiconductor processing and by their unprecedented sensitivity and time response as miniaturized sensing devices [8] , [9] . Unfortunately, as the dimensions of the vibrating structures are reduced to the micro- and nano-scale, their dynamic response at the amplitudes needed for operation frequently becomes nonlinear, with large displacement instabilities and excessive frequency noise considerably degrading their performance [10] , [11] , [12] , [13] . One of the simplest and most popular resonators used in micro- and nano-mechanical resonant sensors and frequency references is the clamped–clamped (c–c) beam resonator [9] , [14] . This type of structure simplifies fabrication at the nanoscale, allows Lorentz force actuation and electromotive detection, and has much higher resonant frequencies than other structures with similar dimensions [9] , [15] , [16] , [17] . On the other hand, a feature usually considered as a disadvantage of c–c beams is that they have a linear response only for oscillation amplitudes that are small compared with their width [18] . This often limits the amplitude at which they are operated, reducing their dynamic range, power-handling capability, and signal-to-noise ratio [19] . Furthermore, when going from micro- to nano-electromechanical systems (MEMS to NEMS), the linear dynamic range can be reduced to the point where the amplitudes needed for lineal response are below the noise level and, as a consequence, operation in the nonlinear regime is unavoidable [20] . In this regime, unlike in the linear one, the resonant frequency has a strong dependence with the oscillation amplitude, an effect similar to what in the quartz literature is known as the amplitude-frequency (a-f) effect [19] , [21] . Because amplitude fluctuations translate into frequency fluctuations, the a-f effect increases considerably the frequency noise of the oscillator and, thus, the benefits of operating at higher amplitudes are undone by the noise increase inherent to operating in the nonlinear regime. Here we address this fundamental limitation by demonstrating a general mechanism for stabilizing the oscillation frequency of nonlinear self-sustaining micro- and nano-mechanical resonators. This is achieved by coupling two different vibrational modes through an internal resonance, where the energy exchange between modes is such that the resonance of one mode absorbs the amplitude and frequency fluctuations of the other, effectively acting as a stabilizing mechanical negative feedback loop. Internal resonance condition in a clamped–clamped beam The dynamics of a c–c beam can be approximated by that of a mass-spring system with a nonlinear restoring force F r =− k 1 x − k 3 x 3 , where x is the displacement of the centre of the beam, k 1 is a linear elastic constant, and k 3 is a nonlinear elastic constant caused by the elongation of the beam as it moves laterally [22] . In the case of damped, harmonically driven oscillations, the equation of movement is then given by the Duffing equation where m eff is the effective mass, c is the damping constant, and F 0 cos( ωt ) is the driving force with amplitude F 0 and frequency f = ω /2π. In the case of a c–c beam, k 3 is positive and the typical resonance curves, calculated by solving equation 1, are shown in Fig. 1a for different driving forces. 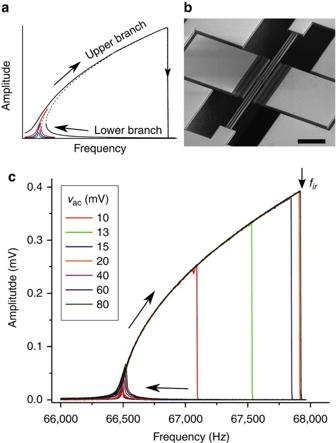Figure 1: Clamped–clamped oscillator and open-loop amplitude resonance curves. (a) Calculated solutions of the Duffing equation. The peak frequency is pulled towards higher frequencies as the driving amplitude is increased (a-f effect). For amplitudes larger than a critical amplitude, the response follows a hysteresis loop, and multivalued regions are formed. When sweeping the driving frequency upwards, the resonant curve will follow the upper branch, up to the peak frequency, where it jumps down, returning through the lower branch. The points represented by the dashed lines are unstable solutions of equation 1 (ref.18). (b) Scanning electron micrograph of a c–c beam resonator with comb-drive electrodes for driving and detection. It is composed of three interconnected beams, of lengthl=500 μm, widthw=3 μm, and thicknesst=10 μm. Scale bar, 100 μm. (c) Measured amplitude resonance curves of the c–c beam resonator withνdc=6 V and different values ofνac. Forνac<20 mV, the peak frequency increases with driving strength, but for the higher driving voltages the peak frequency remains constant atfir∼67,920 Hz, because of the coupling of the first mode with a higher frequency mode through an internal resonance. Figure 1: Clamped–clamped oscillator and open-loop amplitude resonance curves. ( a ) Calculated solutions of the Duffing equation. The peak frequency is pulled towards higher frequencies as the driving amplitude is increased (a-f effect). For amplitudes larger than a critical amplitude, the response follows a hysteresis loop, and multivalued regions are formed. When sweeping the driving frequency upwards, the resonant curve will follow the upper branch, up to the peak frequency, where it jumps down, returning through the lower branch. The points represented by the dashed lines are unstable solutions of equation 1 (ref. 18 ). ( b ) Scanning electron micrograph of a c–c beam resonator with comb-drive electrodes for driving and detection. It is composed of three interconnected beams, of length l =500 μm, width w =3 μm, and thickness t =10 μm. Scale bar, 100 μm. ( c ) Measured amplitude resonance curves of the c–c beam resonator with ν dc =6 V and different values of ν ac . For ν ac <20 mV, the peak frequency increases with driving strength, but for the higher driving voltages the peak frequency remains constant at f ir ∼ 67,920 Hz, because of the coupling of the first mode with a higher frequency mode through an internal resonance. Full size image A scanning electron microscopy image of a typical clamped–clamped oscillator studied in our experiment is presented in Fig. 1b : it consists of interconnected beams with lateral comb-drive electrodes for actuation and detection. In Fig. 1c , we plot several resonance amplitude curves measured with the c–c beam resonator shown in Fig. 1b . All the measurements presented in this work are at room temperature and in vacuum (pressure of 10 −5 mbar). The electrostatic actuation and detection is implemented with lateral capacitive comb-drive electrodes and the driving force is generated by applying an electric voltage ν (t)= ν dc + ν ac sin( ωt ) to one of the comb-drive electrodes, where ν dc is a dc voltage and ν ac is the amplitude of the applied ac voltage. In the four curves corresponding to driving voltages ν ac from 10 to 20 mV, the peak frequency increases with the driving strength, as expected in a Duffing oscillator. In contrast, the curves corresponding to higher driving voltages (40 to 80 mV) all fall to the lower branch at the same frequency f ir =67920 Hz. The reason for this is that, at this frequency, the first mode couples to a higher frequency mode through an internal resonance. This higher frequency mode drains mechanical energy from the first mode reducing its amplitude up to the point where oscillations at that frequency are unstable, thus causing the amplitude to drop to the lower branch of the resonant curve. Since the dominant nonlinearity is cubic this higher frequency mode is expected to have a frequency three times larger than f ir . In this situation a strong interaction between the first and the higher frequency mode is expected and an internal resonance occurs [18] . When applying larger driving voltages ( ν ac >400 mV) the amplitude curve gets across the internal resonance condition without falling to the lower branch, although with a sharp dip at f ir ( Fig. 2a ). 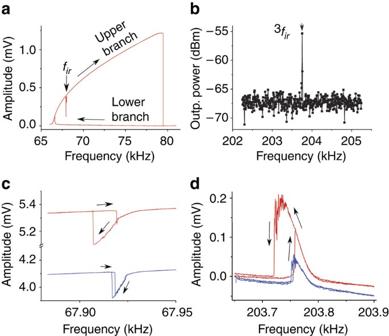Figure 2: Internal resonance in a c–c beam resonator. (a) Resonance curve of the first mode, withνac=2 V andνdc=6 V. There is a sharp dip in the upper branch of the amplitude curve atfir, because, at the internal resonance condition, part of the mechanical energy of the first mode is transferred to a higher frequency mode and, as a result, the amplitude of the first mode is reduced. (b) Accordingly, the resonance of the higher frequency mode at 3firproduces a peak in the output power spectrum (see Methods). No peak is observed in the output power spectrum for driving frequencies different thanfiror when exciting the first mode along the lower branch of the amplitude curve. (c) Detail of the upper branch of the first-mode resonance curve, around the internal resonance condition for aνac=2 V (blue line) andνac=3 V (red line). Here the driving frequency is swept throughfirwhile the oscillation amplitudes of (c) the first mode, and (d) the higher frequency mode, are simultaneously measured with two lock-in amplifiers, with reference signals nearfirand 3fir, respectively. A change in the amplitude of the first mode corresponds to an opposite variation of the amplitude of the higher frequency mode, clearly demonstrating the transfer of mechanical energy between the modes at the internal resonance condition. Figure 2: Internal resonance in a c–c beam resonator. ( a ) Resonance curve of the first mode, with ν ac =2 V and ν dc =6 V. There is a sharp dip in the upper branch of the amplitude curve at f ir , because, at the internal resonance condition, part of the mechanical energy of the first mode is transferred to a higher frequency mode and, as a result, the amplitude of the first mode is reduced. ( b ) Accordingly, the resonance of the higher frequency mode at 3 f ir produces a peak in the output power spectrum (see Methods). No peak is observed in the output power spectrum for driving frequencies different than f ir or when exciting the first mode along the lower branch of the amplitude curve. ( c ) Detail of the upper branch of the first-mode resonance curve, around the internal resonance condition for a ν ac =2 V (blue line) and ν ac =3 V (red line). Here the driving frequency is swept through f ir while the oscillation amplitudes of ( c ) the first mode, and ( d ) the higher frequency mode, are simultaneously measured with two lock-in amplifiers, with reference signals near f ir and 3 f ir , respectively. A change in the amplitude of the first mode corresponds to an opposite variation of the amplitude of the higher frequency mode, clearly demonstrating the transfer of mechanical energy between the modes at the internal resonance condition. Full size image The signal produced by the mode at a frequency 3 f ir can be detected directly by measuring the resonance curve of the first mode while simultaneously monitoring the output power spectrum in the vicinity of 3 f ir . These measurements are presented in Fig. 2 , showing that the dip in the amplitude curve of the first mode ( Fig. 2a ) corresponds to the resonance peak of the higher frequency mode ( Fig. 2b ). Additionally, we see that the hysteresis in the amplitude curve of the first mode ( Fig. 2c ) is also observed in the higher frequency mode resonance curve ( Fig. 2d ), which appears to have a softening nonlinearity. We ran a modal analysis of the resonator with a finite element simulation sofware (Coventorware) to determine which is the mode with natural frequency 3 f ir ∼ ≈203,760 Hz that couples with the first mode at the internal resonance condition ( Fig. 3 ). The simulation shows that, taking into account the tolerance of the fabrication process, two different modes can have this natural frequency: one is the principal flexural out-of-plane mode (mode 2, f ∼ ≈170 KHz), and the other is the principal torsional mode (mode 3, f ∼ ≈230 KHz). These two modes both have an out-of-plane type of motion, and they can both be detected capacitively with the comb drive electrodes. However, in contrast to the case of the first mode, their capacitive variation has twice the frequency of their mechanical oscillations and thus the output signal must be detected at double the frequency of the driving force (2 f detection). Additionally, mode 2 is flexural, like the first mode, and should show a hardening nonlinearity due to the geometry of the clamped–clamped beam, as the first mode does. In contrast, as mode 3 is torsional, it is expected to show a softening nonlinearity, if any, due to the electrostatic potential introduced by the driving and detection electrodes [23] . Therefore, as the mode at 3 f ir shows a softening nonlinearity at high amplitudes, we conclude that it is mode 3 that couples with the first mode at the internal resonance. 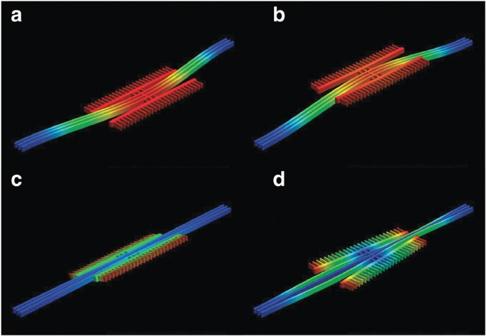Figure 3: Modal analysis of the clamped–clamped beam resonator. Images of the modal displacement of the c–c resonator shown inFig. 1b. The images were obtained using the finite element method simulation software, Coventorware. The calculated resonant frequencies of the different modes are: (a) principal in-plane flexural mode, 68,444 Hz; (b) principal out-of-plane flexural mode, 170,173 Hz; (c) principal torsional mode, 230,108 Hz and (d) in-plane antisymmetric mode: 293,352 Hz. These images are indicative of the dynamic behaviour of the different modes and should not be used to compare relative modal displacement. Figure 3: Modal analysis of the clamped–clamped beam resonator. Images of the modal displacement of the c–c resonator shown in Fig. 1b . The images were obtained using the finite element method simulation software, Coventorware. The calculated resonant frequencies of the different modes are: ( a ) principal in-plane flexural mode, 68,444 Hz; ( b ) principal out-of-plane flexural mode, 170,173 Hz; ( c ) principal torsional mode, 230,108 Hz and ( d ) in-plane antisymmetric mode: 293,352 Hz. These images are indicative of the dynamic behaviour of the different modes and should not be used to compare relative modal displacement. Full size image The experimental results presented in Fig. 2 and the finite element modal analysis of Fig. 3 show that there is a mode at 3 f ir corresponding to the first out-of-plane torsional mode in this device. This mode is expected to show softening nonlinearities due to the electrostatic potential introduced by the driving and detection voltages in the comb drives [23] , in agreement with the experimental data shown in Fig. 2d . In brief, when the first mode is driven along the upper branch of the nonlinear resonant curve with a frequency f ir , an internal resonance occurs. At this frequency, the first mode couples with another mode, with natural frequency 3 f ir , driving it into resonance and resulting in a transfer of mechanical energy between the two modes. The energy exchange between modes is such that, if the amplitude of the second mode increases, it draws energy from the first mode and thus decreases its amplitude. Similarly, if the amplitude of the second mode decreases, then the amplitude of the first mode is increased. Amplitude and frequency stabilization The energy transfer between modes described in the previous section has a direct impact on the amplitude stability of the first mode and can be used as a mechanical negative feedback to stabilize both its amplitude and frequency. To qualitatively understand how this works, let's assume that the resonator is in the internal resonance condition, with the first mode oscillating in the upper branch of the resonance curve and the higher frequency mode oscillating just below its resonant frequency at 3 f ir , driven by the oscillations of the first mode. At this point, if fluctuations increase the amplitude of the first mode, then its frequency also increases owing to the a-f effect. This drives the higher frequency mode oscillation closer to the peak of its resonance, and thus its amplitude increases. As a result, more energy is drawn from the first mode, decreasing its amplitude and frequency, thus effectively opposing the increase in amplitude and frequency produced by noise. On the other hand, if the amplitude of the first mode decreases, then its frequency also decreases. This moves the frequency of the higher frequency mode oscillation away from the resonance peak, thus decreasing its amplitude. Consequently, less energy is drawn from the first mode and its amplitude and frequency increase. In other words, the higher frequency mode is effectively stabilizing the amplitude and frequency fluctuations of the first mode. A simple theoretical description of the proposed stabilization mechanism can be obtained by introducing a coupling term into the Duffing equation, equation 1, and by adding a second equation describing the high-frequency mode dynamics. This simple set of equations can be solved analytically, providing a convincing theoretical analysis for the negative feedback effect responsible for stabilizing the oscillator's frequency ( Supplementary Figure S1 ). This model for the dynamics of the modes and their interaction is presented in the Supplementary Methods . To verify experimentally this internal mechanical stabilization mechanism, we drive the resonator in a closed loop configuration, where the oscillations are self-sustained at ∼ 500 Hz below f ir ( Fig. 4a ). Then we start increasing ν ac to reach the internal resonance condition, and for each value of ν ac we measure the frequency of oscillations as a function of time for 120 s, using an averaging time of 0.1 s for each point. From these measurements, we calculate the mean frequency and the standard deviation of the frequency as a function of ν ac . 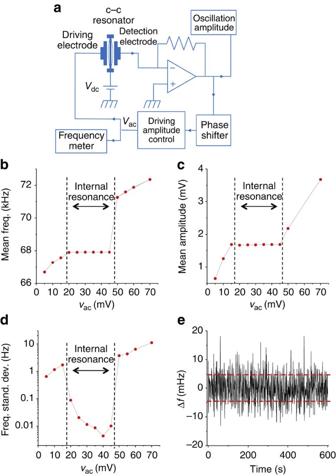Figure 4: Frequency stabilization of the self-sustaining oscillator. (a) Circuit schematic of the c–c resonator in a closed loop configuration that maintains the self-sustained oscillations (see Methods). (b) Mean frequency of the first-mode oscillations. The frequency versus driving amplitude curve flattens, when the internal resonance condition is reached atfir. (c) Amplitude of the first-mode oscillations. Similarly to what happens to the frequency, the amplitude versus driving force curve flattens when the internal resonance condition is reached atfir. The amplitude in millivolts may differ from that of the open loop curves ofFig. 1cowing to different settings in the current preamplifier and lock-in amplifier gains. (d) Standard deviation of the self-sustaining oscillator's frequency (on a logarithmic scale), showing how the frequency fluctuations are substantially reduced, once the internal resonance condition is reached. (e) Frequency variation Δf=f−fmeanat the internal resonance condition (fmean=fir), measured using an averaging time of 0.1 s. Through an interval of 600 s, the standard deviation of the frequency, measured in units of parts per million, is 0.06 p.p.m. (red lines), whenνac=40 mV. All the measurements are at room temperature and in a vacuum of 10−5mbar. Figure 4: Frequency stabilization of the self-sustaining oscillator. ( a ) Circuit schematic of the c–c resonator in a closed loop configuration that maintains the self-sustained oscillations (see Methods). ( b ) Mean frequency of the first-mode oscillations. The frequency versus driving amplitude curve flattens, when the internal resonance condition is reached at f ir . ( c ) Amplitude of the first-mode oscillations. Similarly to what happens to the frequency, the amplitude versus driving force curve flattens when the internal resonance condition is reached at f ir . The amplitude in millivolts may differ from that of the open loop curves of Fig. 1c owing to different settings in the current preamplifier and lock-in amplifier gains. ( d ) Standard deviation of the self-sustaining oscillator's frequency (on a logarithmic scale), showing how the frequency fluctuations are substantially reduced, once the internal resonance condition is reached. ( e ) Frequency variation Δ f = f − f mean at the internal resonance condition ( f mean = f ir ), measured using an averaging time of 0.1 s. Through an interval of 600 s, the standard deviation of the frequency, measured in units of parts per million, is 0.06 p.p.m. (red lines), when ν ac =40 mV. All the measurements are at room temperature and in a vacuum of 10 −5 mbar. Full size image For driving voltages lower than 20 mV, the mean frequency and the oscillation amplitude increase with voltage ( Fig. 4b,c ), as expected in a Duffing resonator. In this driving range, the noise in the frequency also increases with voltage ( Fig. 4d ), because the oscillator becomes more nonlinear and thus the a-f effect increases. At ν ac =20 mV, both the frequency and the amplitude values levels off and remain constant as ν ac is further increased ( Fig. 4b,c ). This is the onset of the internal resonance condition, where the high-frequency mode couples with the first mode and stabilizes both its amplitude and frequency of oscillation. Consequently, as shown in Fig. 4d , the frequency fluctuations drop substantially, from 1.75 Hz to 4 mHz at ν ac =40 mV, almost 400 times, giving a frequency stability In Fig. 4e , we plotted the instantaneous frequency variation versus time curve for ν ac =40 mV, showing the excellent frequency stability over times of several minutes. The short-term frequency fluctuation of our oscillator, working deep in the nonlinear regime, is comparable to state-of-the-art MEMS/NEMS linear oscillators [9] , [24] , [25] . When the driving amplitude is further increased, the end of the internal resonance condition is reached. At that point, the high-frequency mode stops opposing the amplitude and frequency increase of the first mode, and the frequency jumps to the value expected for the Duffing resonator. Additionally, as the stabilizing action of the high-frequency mode is no longer in effect, the frequency noise increases abruptly. Additional information about the frequency noise can be obtained by analysing the Allan deviation outside and inside the internal resonance condition. In Fig. 4d , the stabilization mechanism is demonstrated by measuring the standard deviation of the frequency, as the driving voltage is increased and the oscillator enters the internal resonance condition. A more complete description of the noise in the oscillator is given by the fractional frequency fluctuations averaged over an interval τ , as a function of that averaging time τ . This is known as the Allan deviation σ y ( τ ) and can be expressed as where are the relative frequency fluctuations averaged over the i th discrete time interval of τ . In Fig. 5a, we show the Allan deviation of the oscillator at the internal resonance condition ( ν ac =40 mV). It can be observed that the behaviour of the curve is as expected in a mechanical oscillator: for short averaging times, the deviation diminishes with the averaging time (up to ∼ 10 s), because the fluctuations are dominated by white noise, and for longer times the deviation increases with averaging time, because the noise process is dominated by random walk of frequency. In Fig. 5b , we show the Allan deviation for the oscillator inside ( ν ac =40 mV) and outside ( ν ac =15 mV) the internal resonance condition, clearly showing the frequency stabilization obtained with this mechanism. 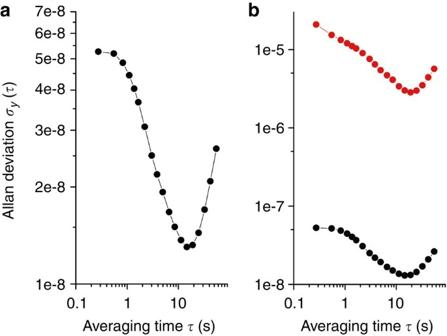Figure 5: Allan deviation of the micromechanical oscillator. (a) Inside the internal resonant condition (νac=40 mV), showing a white noise type for averaging times up to 10 s, and random walk frequency noise for higher averaging times. (b) Outside (νac=15 mV) and inside (νac=40 mV) the internal resonance condition, showing the effect of the stabilization mechanism. Figure 5: Allan deviation of the micromechanical oscillator. ( a ) Inside the internal resonant condition ( ν ac =40 mV), showing a white noise type for averaging times up to 10 s, and random walk frequency noise for higher averaging times. ( b ) Outside ( ν ac =15 mV) and inside ( ν ac =40 mV) the internal resonance condition, showing the effect of the stabilization mechanism. Full size image The frequency noise is induced by undesired forces that affect both the amplitude and, through the a-f effect, the frequency of the oscillations. Examples of these forces are the noise in the driving voltage, variations in pressure and temperature, random vibrations and/or contamination of the resonator element. The internal resonance mechanism reduces the sensitivity of the oscillation amplitude to all of these force fluctuations. If additional stabilization methods are used, such as temperature compensation, then the effects of reducing the noise in the external forces and of using the internal resonance stabilization will be additive. The former will reduce the fluctuations in the forces affecting the oscillation amplitude and the latter will reduce the sensitivity of the oscillation amplitude to these fluctuations. The method presented in this work, for stabilizing the frequency of oscillation through the coupling of modes in the internal resonance condition, could be applied to a wide range of micro- and nano-mechanical oscillators. We observed, in other similar resonators, that the coupling can be obtained not only with the torsional mode but also with the out-of-plane flexural mode ( Supplementary Fig. S2 ), which makes the design easy to implement in c–c beam resonators. For instance, in a single c–c beam with length l , width w and thickness t , the resonant frequency of the first flexural mode that oscillates in the direction of w is (ref. 26 ), where E is the Young modulus, ρ is the density of the beam, and L is the length of the beam. Similarly, the mode that oscillates in the direction of t has a resonant frequency and thus ω 2 / ω 1 = t / w . Therefore, to obtain an internal resonance, we just need that t >3 w so that ω 2 >3 ω 1 and thus, by driving the first mode with an appropriate force, the first mode can be made to resonate at a frequency equal to (1/3) ω 2 . Using the fact that at the internal resonance condition, the peak frequency satisfies f p ( ν ac )= f ir , the value of ν ac needed to achieve the internal resonance conditions can be predicted. The limitations in the driving force and in the attainable frequency detuning of the first mode will set the upper limit for the difference between ω 1 and (1/3) ω 2 . This reasoning holds independently of the frequency or size of the resonator and thus this stabilization method could in principle be applied to high-frequency MEMS and NEMS, in which the linear dynamic range imposes severe limitations to the signal-to-noise ratio, allowing large displacements with excellent frequency stability. To verify this, future experiments should focus on applying the stabilization method to high-frequency nanoscale resonators. In conclusion, we presented a frequency stabilization mechanism that is intrinsic to self-sustained micromechanical resonators operating in the nonlinear regime. This mechanism provides a new strategy for further optimization and engineering of micro- and nano-scale devices and demonstrates that very low-frequency noise performance is possible in the nonlinear regime. The most straightforward application of this mechanism will be in the broad field of miniaturized mechanical oscillators for frequency references, but it can also be used in frequency-shift-based detectors. For this, the same configuration showed here should be used. With the first mode stabilized at f ir , the device is sensitive to variations in the resonant frequency of the higher frequency mode, induced, for example, by changes in mass or force. This is so because these variations modify the value of f ir and thus the frequency of the self-sustained oscillations of the low frequency mode. In this way, the resonant frequency of the high-frequency mode, which is linear and has good stability but has low amplitude, could be followed by detecting the nonlinear low frequency mode, which has a much larger amplitude, increasing the signal-to-noise ratio. Finally, further applications of the internal resonance phenomenon in MEMS and NEMS can be imagined, such as in mechanical energy storage with resonators [27] , where energy input at low frequencies could be stored in higher frequency modes, thus using the multiple degrees of freedom of the resonator to extend its energy storage capacity. Amplitude detection of the two coupled modes Both modes were measured capacitively with the same comb-drive electrodes. The first mode is the principal in-plane flexural mode, and the capacitance variation of the electrodes has the same frequency than the mechanical oscillations. The higher frequency mode is the principal out-of-plane torsional mode and, in this case, the capacitance variation has twice the frequency of the mechanical oscillations. Consequently, while the driving frequency is swept in the vicinity of the internal resonance frequency f ir ¸ the spectrum analyser frequency span is centred at 6 f ir . In this way, the output spectrum corresponding to the oscillations of the higher frequency mode at 3 f ir are detected. In order to simultaneously measure both coupled modes with two different lock-in amplifiers, a reference signal near 6 f ir is used for the high-frequency lock-in to detect the oscillations of the higher frequency mode at 3 f ir . This reference signal is also input into a frequency divider by six and used as the reference for the low frequency lock-in, in the vicinity of f ir . Additionally, this signal is used to drive the resonator and sweep the resonance curve of the first mode around f ir . MEMS resonator detection and actuation The motion of the resonator is detected capacitively. The capacitance variation of the voltage-biased comb-drive electrode generates a current that is introduced into a current amplifier. This amplifier produces a voltage output, proportional to the oscillation amplitude, which is first phase shifted with an active analogue implementation of an all-pass filter and then used as input of the phase-locked loop in the lock-in amplifier (external reference input). The reference output of the lock-in amplifier is phase locked to the input reference, and its amplitude is set by the internal function generator to the specified value. Thus, the resulting signal at the output of the phase-locked loop is phase locked to the detection signal but phase shifted and with a constant amplitude that can be set independently of the amplitude of the oscillations. This resulting signal is used to drive the resonator and to measure the frequency of the oscillations with a digital frequency counter. The phase shift between the excitation and the detection signal determines the point in the resonance curve, where the resonator is phase-locked. For instance, to operate the oscillator in the peak of the resonance curve, the phase shift must be set to − π /2. This is the working point that we used because, for a given driving strength, the amplitude of oscillation is maximum. How to cite this article: Antonio D. et al . Frequency stabilization in nonlinear micromechanical oscillators. Nat. Commun. 3:806 doi: 10.1038/ncomms1813 (2012).